Mirror neurons in monkey area F5 do not adapt to the observation of repeated actions Repetitive presentation of the same visual stimulus entails a response decrease in the action potential discharge of neurons in various areas of the monkey visual cortex. It is still unclear whether this repetition suppression effect is also present in single neurons in cortical premotor areas responding to visual stimuli, as suggested by the human functional magnetic resonance imaging literature. Here we report the responses of ‘mirror neurons’ in monkey area F5 to the repeated presentation of action movies. We find that most single neurons and the population at large do not show a significant decrease of the firing rate. On the other hand, simultaneously recorded local field potentials exhibit repetition suppression. As local field potentials are believed to be better linked to the blood-oxygen-level-dependent (BOLD) signal exploited by functional magnetic resonance imaging, these findings suggest caution when trying to derive conclusions on the spiking activity of neurons in a given area based on the observation of BOLD repetition suppression. It is well established that the repetition of identical visual stimuli results in a decrease of the responses of single neurons in a variety of areas in monkey visual cortex. They include area V1(ref. 1 ), extrastriate visual areas [1] , [2] , [3] , [4] , as well as areas in the inferior [5] , [6] , [7] , [8] , [9] , [10] , [11] , [12] , [13] , [14] , [15] and the medial temporal lobe [16] , [17] , [18] . This response decrease has been varyingly called ‘adaptation’ [18] or ‘repetition suppression’ [19] . The possibility to use adaptation to discover specific visual characteristics in human functional magnetic resonance imaging (fMRI) studies has renewed interest in this phenomenon [1] , [20] , [21] . This fresh interest has also motivated recent studies, mostly focusing on the inferior temporal (IT) lobe, to understand the mechanism and the limits of the adaptation technique in fMRI studies of the human brain [8] , [9] , [12] , [14] . These studies have suggested that adaptation in IT may either depend on a decrease of synaptic efficacy of the afferents carrying visual information to temporal lobe neurons [8] , [12] or it might be the result of improved predictions of experienced visual stimuli (that is, a top–down effect), leading to decreasing prediction errors [22] , [23] , [24] . Yet, recent observations on visual neurons recorded from IT cortex of anesthetized [11] as well as of awake behaving monkeys [9] have not been able to lend support to this latter hypothesis. Conceptually, an interesting question is whether adaptation to visual stimulation is confined to visual neurons located in striate and extrastriate visual cortex or whether it also pertains to neurons outside it, such as, for example, motor areas. Unfortunately, pertinent single neuron data on this issue are limited to prefrontal cortical areas. For these areas, some studies reported a decrease of the neuronal responses to sequences of identical stimuli [25] , others a response increase [14] , [26] , [27] . It should be noted, however, that these findings are difficult to interpret because, typically, response increases were found in cognitive tasks in which the monkeys had to keep the first stimulus in mind to respond correctly to the second one (‘delayed paired associate’ or ‘match to sample’ tasks). The fMRI adaptation technique has recently been employed to reveal the presence of action-responsive (object grasping) neurons in the intraparietal sulcus [28] and, moreover, for studying mirror neurons in the action observation/action execution human network [29] , [30] , [31] , [32] , [33] . The results have been in some cases contradictory and difficult to interpret (see Discussion ). Arguably, this lack of clarity of the effects of stimulus repetition on the responses of single mirror neurons might be a repercussion of the complex integration of motor, sensory and cognitive signals these neurons perform. Unfortunately, to date there is no information on the consequences of repetitive stimulation on the responses of mirror neurons, that could facilitate the interpretation of the fMRI findings. Traditionally, in mirror neuron studies, visual responses have been evoked by actions performed by the experimenter in front of the monkey [34] , [35] . Yet, the inevitable variability of these ‘naturalistic action stimuli’ has made them unsuitable for repetition suppression studies. However, we have recently established that F5 mirror neurons respond not only to ‘naturalistic’ stimuli, but also to filmed actions [36] . Hence, we could use a well-controlled stimulus, namely the repeated presentation of one and the same filmed action, lacking any variability, to reveal changes in neuronal activity. Using this approach in this study, we found that most mirror neurons and the population at large did not show a significant decrease of their firing rate. On the other hand, simultaneously recorded local field potentials (LFPs), believed to be better linked to the blood-oxygen-level-dependent (BOLD) signal, exhibited repetition suppression. Effects of observing a repeated action on mirror neurons We recorded 785 neurons from area F5 of two rhesus monkeys ( Macaca mulatta ). Of these neurons, 632 discharged in association with the monkey’s hand grasping an object; 247 were also active during the observation of the same motor act when presented in a movie on the monitor in front of the monkey and therefore identified as mirror neurons. In about 20% of the trials that will be referred to as ‘test trials’ the monkeys saw a movie ( Fig. 1a ) that started with the presentation of an object (a pepper). Then a hand entered the scene, reached out for the object, grasped it without moving it and finally withdrew without the object. The movie ended with the pepper left on the screen. After 640 ms the same movie was presented again. The other 80% of trials involved different types of hand-object interactions or, alternatively, interactions between two non-biological objects, which in human observers typically evoke a percept of causality. The size of the set from which these different types of ‘non-test trials’ were chosen varied from 5 to 11, depending on the particular experiment. In these ‘non-test trials’, a given movie was either followed by repeated presentation of the same or by a presentation of a different movie (90% of the cases). To assess whether the repeated presentation of the same action led to a change of the discharge of a mirror neuron, we considered only test trials. The reason to deploy test trials with the particular type of object-related motor act sketched before was that a preceding exploration of F5 had clearly demonstrated that mirror neurons in the region exploited for the present study were typically sensitive to it. In accordance with the well-established characteristics of mirror neurons [34] , [36] , [37] , all the mirror neurons in our sample preferred goal-directed motor acts over non-goal-directed motor acts or the occurrence of an object (see Methods for details). 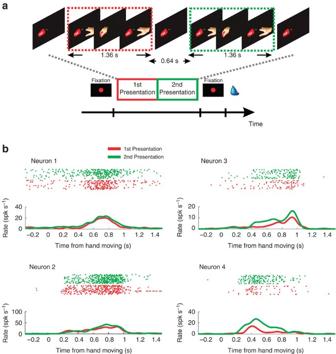Figure 1: Test stimuli and exemplary single neurons. (a) Schematic illustration of a trial. The movie started with the presentation of an object, followed by a reaching motor act. After about 640 ms the identical movie was repeated. (b) Examples of single-unit responses of mirror neurons evoked by the first and the second presentation of the action movie. Neurons 1 and 2 are two examples of neurons with no difference in response strength when the action was repeated. Neurons 3 and 4 are two examples of neurons in which the response to the second presentation of the action was significantly stronger than the response to the first one. Figure 1: Test stimuli and exemplary single neurons. ( a ) Schematic illustration of a trial. The movie started with the presentation of an object, followed by a reaching motor act. After about 640 ms the identical movie was repeated. ( b ) Examples of single-unit responses of mirror neurons evoked by the first and the second presentation of the action movie. Neurons 1 and 2 are two examples of neurons with no difference in response strength when the action was repeated. Neurons 3 and 4 are two examples of neurons in which the response to the second presentation of the action was significantly stronger than the response to the first one. Full size image Figure 1b shows the responses of four mirror neurons to the presentation of a first (red) and a second (green) action movie. Neurons 1 and 2 are examples of neurons whose responses were identical during the first and the second presentation. Neurons 3 and 4 are examples of neurons in which the second movie evoked a stronger response than the first one. Out of the 247 mirror neurons responding to the presentation of the test stimulus (see Supplementary Table S1 ), 163 (66%) did not show a significant change of their discharge from the first to the second presentation of the action movie, whereas such a change was found in the remaining 84 (34%, P <0.05, sign-rank test). However, in contrast to our expectation, the majority of these neurons exhibited a significant increase of their response ( n =55) rather than a decrease ( n =29). 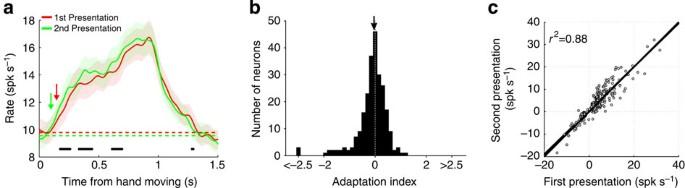Figure 2: Analysis of population response based on all mirror neurons in the sample. (a) Population response (n=247) as function of time for the first (red) and the second (green) presentation of the action. The continuous coloured line is the average and the shaded region the s.e.m. Arrows (red=144 ms—first presentation, green=106 ms—second presentation) indicate the onset of the response identified as points at which the discharge exceeded the average activity of the first 80 ms (dashed line) following the beginning of the hand-moving action (P<0.05, sign-rank test). The black horizontal line indicates the period of time in which the two populations were different (P<0.05, running sign-rank test). (b) Distribution of adaptation indices. The index is given by the difference between the average activity evoked by the first minus the average activity evoked by the second presentation of the action normalized by the average activity evoked by the first presentation. Averages are based on the period of time in which the hand was moving towards the object until, when withdrawing from the object, the hand exited the scene. (c) Scatter plot of the average activity during the first presentation as function of the activity during the second presentation of the visual stimulus. Data were fitted with a linear regression model (see text for further details). Figure 2a shows the averaged non normalized population spike density functions for the two presentations. The responses were similar in the two cases most of the time ( Fig. 2a ; P <0.05, running paired sign-rank test). There were, however, short time periods in which the responses were actually stronger during the second presentation ( Fig. 2a , horizontal lines). A small but significant increase of the response due to repetition is also revealed by considering the distribution of the sample ‘adaptation index’ [8] . This index results from subtracting the average activity evoked by the second action presentation from the average activity evoked by the first one, normalized by dividing the difference by the average activity of the first presentation. The index is 0 for identical responses. Figure 2b shows the distribution of the adaptation index for the present data. The index is slightly—but significantly—shifted towards negative values reflecting stronger responses to the second presentation (median=−0.04, P =0.029; sign-rank test against median 0). Moreover, the absence of adaptation was independent on the specific choice of the index ( Supplementary Table S2 ). Figure 2: Analysis of population response based on all mirror neurons in the sample. ( a ) Population response ( n =247) as function of time for the first (red) and the second (green) presentation of the action. The continuous coloured line is the average and the shaded region the s.e.m. Arrows (red=144 ms—first presentation, green=106 ms—second presentation) indicate the onset of the response identified as points at which the discharge exceeded the average activity of the first 80 ms (dashed line) following the beginning of the hand-moving action ( P <0.05, sign-rank test). The black horizontal line indicates the period of time in which the two populations were different ( P <0.05, running sign-rank test). ( b ) Distribution of adaptation indices. The index is given by the difference between the average activity evoked by the first minus the average activity evoked by the second presentation of the action normalized by the average activity evoked by the first presentation. Averages are based on the period of time in which the hand was moving towards the object until, when withdrawing from the object, the hand exited the scene. ( c ) Scatter plot of the average activity during the first presentation as function of the activity during the second presentation of the visual stimulus. Data were fitted with a linear regression model (see text for further details). Full size image To exclude that the large number of trials may not have concealed adaptation effects associated with a few early action stimuli, we calculated the adaptation indices based on the first trials of a given session (using alternatively the first, the first two or the first three trials) and compared them with the ones obtained for the last trials (correspondingly using the last trial, the last two or the last three trials). As the distributions of the ‘early’ adaptation indices were not different from the ‘late’ ones (for all of them P >0.05, sign-rank test; first one versus last one median=0, first two versus last two median=−0.009, first three versus last three median=0), a ‘familiarity’ effect does not appear to be a valid explanation of a lack of significant adaptation. Finally, a slight shift towards negative values (reflecting an increase of the activity with repetition) was also obtained when the adaptation index calculated for complete sessions was based on measures of maximum peak activity rather than average activity (index calculated as maximum absolute net activity during the first presentation minus the maximum absolute net activity during the second presentation, normalized by the maximum absolute net activity during the first presentation; median=−0.003, P =0.022; sign-rank test against median 0). On the other hand, a simple regression of the average responses to the second action presentation, as function of the average responses to the presentation of the first action, ( Fig. 2c ) was not sensitive enough to reveal the weak increase of the activity as indicated by the fact that the regression did not significantly differ from the diagonal (bootstrapped confidence intervals at P =0.05: slope=[0.817 1.061], intercept c =(−0.045 0.953)). To reveal possible changes of the timing of the responses to the second as compared with the first presentation, we cross-correlated the spike density functions of individual neurons for the whole duration of the first and the second presentation and identified the lag of the maximum of the resulting cross-correlation function. The mean lag was not different from 0 ( P >0.05, sign-rank test against median 0) indicating that the repetition of the stimuli did not lead to systematic time shifts of the response profiles. The lack of repetition suppression observed might reflect the cancellation of adaptation due to putative facilitatory influences counteracting it. One potentially relevant process might be the allocation of attention as reflected by the pattern of fixations and saccades made when scrutinizing the action stimuli. To address this possibility, we analysed the eye fixation pattern of the monkeys during the presentation of the movies. However, as described in detail in Supplementary Note 1 , we were neither able to find any relevant differences in fixation patterns between the first and the second presentation of the action stimulus, nor could we detect any influence of eye position or eye movements on the neuronal discharge. A second potential confound to consider is the effect of reward. A reward was given at the end of the fixation period, which ranged from 0.5 to 1.5 s following the presentation of the second action stimulus (see Fig. 1a and Supplementary Fig. S1 ). Hence, one might argue that the expectation of the reward might have led to a response increase following the second presentation of the action stimuli. Actually, the analysis revealed that indeed 35% of the tested neurons showed a significant increase of their discharge in the period following the end of the second action stimulus, when the monkey was waiting for the delivery of the reward. Although the onset of this reward-related discharge increase followed the end of the second movie with a clear delay, a preparatory state, modifying the preceding visual response is, in principle, impossible to exclude. However, a strong argument against this interpretation is the finding that the neurons that showed a significant reward-related discharge increase and those that did not show it, did not differ in their adaptation indices ( n =160 neurons without significant reward-related response, average adaptation index −0.045, max adaptation index −0.003; n =87 with reward response, average adaptation index −0.047, max adaptation index −0.003, difference P >0.5, U -test; the average adaptation index activity of the reward-responsive neurons was not correlated with the reward-related activity, P >0.1, Spearman correlation, see Supplementary Fig. S2 ). This latter analysis clearly speaks against an influence of reward expectancy. Yet, to rule out the reward expectancy hypothesis more firmly, we carried out a second experiment. Effects of observing a fourfold action on mirror neurons In Experiment 2, we presented the same action stimuli as in Experiment 1, but with four repetitions rather than two (see Methods ). By using this procedure, reward expectancy, building up at the end of the four stimuli sequence, was well separated in time from the first two presentations of the action stimuli. The inclusion criteria for neurons investigated in this experiment were the same as those used in the main experiment. Fifty neurons, recorded from one monkey, were tested. 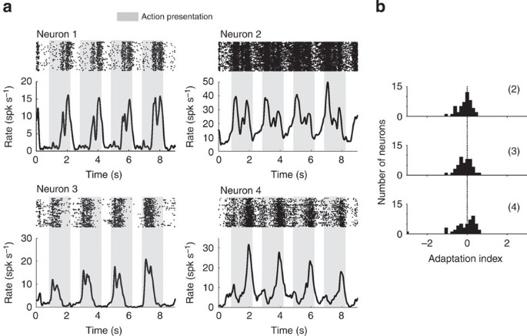Figure 3: Repetition of four identical actions. (a) Examples of four mirror neurons exhibiting responses associated with the observation of a sequence of four identical object-related hand actions. The grey background indicates the period in which the human hand was reaching for the pepper, grasping it—however, without moving it—and ultimately being withdrawn from it. (b) Distributions of adaptation indices comparing responses to the second (2), third (3) and fourth (4) action stimulus, respectively, with the first one. The distributions of adaptation indices are based onn=50 mirror neurons tested in the control experiment. The fact that the distributions are centred on 0 (see text), indicates the absence of any consistent effect of stimulus repetition at the population level. Figure 3a shows the responses of four neurons to the sequence of four action presentations. Neurons 1 and 2 (upper row) did not show any significant difference between the responses to the four presentations. Neuron 3 showed a progressive response increase, whereas Neuron 4 exhibited a response decrease. Figure 3: Repetition of four identical actions. ( a ) Examples of four mirror neurons exhibiting responses associated with the observation of a sequence of four identical object-related hand actions. The grey background indicates the period in which the human hand was reaching for the pepper, grasping it—however, without moving it—and ultimately being withdrawn from it. ( b ) Distributions of adaptation indices comparing responses to the second (2), third (3) and fourth (4) action stimulus, respectively, with the first one. The distributions of adaptation indices are based on n =50 mirror neurons tested in the control experiment. The fact that the distributions are centred on 0 (see text), indicates the absence of any consistent effect of stimulus repetition at the population level. Full size image A direct comparison of the first and second presentation of the goal-directed motor act revealed that out of the 50 mirror neurons tested, 31 (62%) did not show any significant response change, whereas 19 (38%) exhibited a change of their action-related discharge ( P <0.05, sign-rank test). Of these, 14 neurons exhibited responses to the second presentation that were stronger than that to the first presentation, whereas only in five neurons the opposite was found. At the population level, average activities for the four repetitions were not different (see Supplementary Fig. S3 , Friedman’s test, P >0.05 with subsequent post-hoc comparisons based on sign-rank tests, Bonferroni corrected). Figure 3b displays the distributions of adaptation indices of the second (2), third (3) and fourth (4) action presentation relative to the first one (sign-rank test against median 0: second presentation median=−0.0176, P =0.0566; third presentation median=−0.0952, P =0.0249; fourth presentation median=0.0568, P =0.7751). These findings are in accordance with those of Experiment 1, indicating the absence of any consistent adaptation effect due to stimulus repetition at the population level. A regression analysis (not shown) comparing the spike rates of the second versus the first presentation resulted in a highly significant fit ( r 2 =0.93, P <0.05) with the regression line not differing significantly from the diagonal (bootstrapped confidence intervals at P =0.05: slope (0.833 1.186), intercept c =(−0.563 0.950)). Also in this case the neurons showing or not showing a significant reward-related discharge increase did not differ in their adaptation indices ( n =15 neurons without significant reward-related response, median of the average adaptation index=−0.017, median of the maximal adaptation index=−0.051; n =39 with reward-related response, median of the average adaptation index=−0.001, median of the maximal adaptation index=−0.027, difference P >0.5, U -test; the average adaptation index activity of the reward-responsive neurons was not correlated with the reward-related activity, P >0.1, Spearman correlation). Effects of observing a repeated action on LFPs As it has been suggested that BOLD activity could be more correlated with LFP than with single neurons output, we—in addition to the analysis of the single neuron responses during the adaptation paradigm—also studied the simultaneously recorded LFP activity. Action-related evoked LFP records were isolated by band pass filtering (1–100 Hz, see methods for details) the signals extracted from the same electrodes used to record the action potentials of mirror neurons discussed in Experiment 1. Average evoked LFP responses were calculated for each individual session and they were aligned, as for mirror neurons action potentials, with respect to the beginning of the first and the second-hand motor act, respectively ( Methods ). 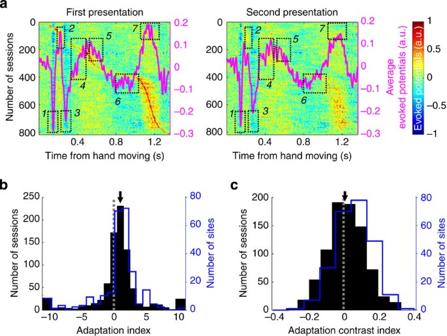Figure 4: Analysis of population response of the LFPs. (a) Population response (n=819 session) as function of time for the first (left column) and the second (right column) presentation of the action. Same time events as inFigs 1and2. The colour plot in the background shows all the single sessions (sorted with respect to the time of maximum response for graphical purposes) whereas the pink continuous coloured line gives the median activity. Dashed rectangles indicates regions in which the activity over time showed either repetition suppression (1,2,3,5,6 and 7) or enhancement (4). (b) Distribution of adaptation indices for all sessions (black) and for the reduced set of recording sites (blue, seeMethods). The index is given by the difference between the average activity evoked by the first minus the average activity evoked by the second presentation of the action normalized by the average activity evoked by the first presentation. Averages are based on the period of time in which the hand was moving towards the object until, when withdrawing from the object, the hand exited the scene. Positive value of this index indicates the reduction of the activity of the second presentation when compared with the first (median=0.778,P<0.001 sign-rank test). (c) Distribution of adaptation contrast indices. The index computes the difference between the square root of the arithmetic sum of the squares of the first minus the second presentation divided by their sum. Positive value of this index indicates the reduction of the activity of the second presentation when compared with the first (median=0.018,P<0.001, sign-rank test). Figure 4a shows all the LFPs recorded in the single sessions (in the background) and the grand average LFP response for all the sessions available (in the foreground in pink). The average LFP response consisted of a sequence of multiple peaks. As indicated by a running sign-rank test ( P <0.05) seven of them, marked by dashed squares in Fig. 4a , deviated significantly from baseline. The amplitudes of these peaks were smaller for the second presentation, a suppression that was significant for all except for peak 4 (Friedman’s test, P <0.05 with subsequent post-hoc comparisons based on sign-rank tests, Bonferroni-corrected). Figure 4: Analysis of population response of the LFPs. ( a ) Population response ( n =819 session) as function of time for the first (left column) and the second (right column) presentation of the action. Same time events as in Figs 1 and 2 . The colour plot in the background shows all the single sessions (sorted with respect to the time of maximum response for graphical purposes) whereas the pink continuous coloured line gives the median activity. Dashed rectangles indicates regions in which the activity over time showed either repetition suppression (1,2,3,5,6 and 7) or enhancement (4). ( b ) Distribution of adaptation indices for all sessions (black) and for the reduced set of recording sites (blue, see Methods ). The index is given by the difference between the average activity evoked by the first minus the average activity evoked by the second presentation of the action normalized by the average activity evoked by the first presentation. Averages are based on the period of time in which the hand was moving towards the object until, when withdrawing from the object, the hand exited the scene. Positive value of this index indicates the reduction of the activity of the second presentation when compared with the first (median=0.778, P <0.001 sign-rank test). ( c ) Distribution of adaptation contrast indices. The index computes the difference between the square root of the arithmetic sum of the squares of the first minus the second presentation divided by their sum. Positive value of this index indicates the reduction of the activity of the second presentation when compared with the first (median=0.018, P <0.001, sign-rank test). Full size image To better quantify the overall decrease, we calculated adaptation indices for individual sessions by subtracting the average activity of the LFPs evoked by the second action presentation from the average activity of the LFPs evoked by the first one, normalized by dividing the difference by the average activity of the LFPs of the first presentation. In accordance with the visual impression conveyed by the grand average LFP response, the distribution of the resulting adaptation indices were significantly shifted towards positive values ( Fig. 4b ), indicating clear repetition suppression (median=0.778, P <0.01, sign-rank test). We further compared the responses by computing an ‘adaptation contrast index’ (see Methods ), based on the difference between the squared root of the sum of the squared LFPs evoked by the first presentation minus the squared root of the sum of the squared LFPs evoked by the second presentation and then dividing this difference by the sum of the squared LFPs evoked by the first presentation plus the squared root of the sum of the squared LFPs evoked by the second presentation (see Methods for details). This measure, which has the advantage of eliminating the influence of the sign of LFP response components, similarly demonstrated a significant suppression ( Fig. 4c ). This was indicated by a median of the distribution that significantly deviated from zero (median=0.018, P <0.05, sign-rank test). The aim of the present study was to examine the effect of stimulus repetition on the responses of mirror neurons in premotor area F5. The results show that the majority of mirror neurons do not exhibit adaptation of their responses to the repeated presentation of an action. Only few of them showed a response decrease, whereas a substantial number exhibited an increase of their responses. Most importantly, the population, as a whole, displayed a significant, albeit slight, increase in response strength following stimulus repetition. On the other hand, the evoked LFPs recorded together with mirror neuron action potentials exhibited clear repetition suppression. It is important to note that we tested mirror neurons in a pure observation task, in which no memory of the previously presented stimulus was required. This allowed us to rule out the possibility that the facilitatory effect we observed at the population level was due to memory-related factors as in experiments in which ‘delayed paired associate’ or ‘match to sample’ tasks were used [14] , [26] , [27] . Another factor that could have, in principle, counteracted adaptation is reward expectancy. However, this possibly confounding factor was ruled out by the analysis of the background activity in Experiment 1 and, more specifically by Experiment 2, in which we examined neuronal responses to sequences of four repeated identical action stimuli. Also in this experiment no adaptation was present. The lack of adaptation of the observation-related responses of F5 mirror neurons seems to contradict the overwhelmingly consistent demonstration of repetition suppression of BOLD responses [28] , [31] , [38] , [39] , [40] evoked by the observation of actions from parts of human frontal cortex thought to represent a homologue of monkey area F5 [41] , [42] . The only exception is a report by Lingnau et al. [33] , who, when showing intransitive actions to subjects, did not observe significant repetition suppression of BOLD activity in areas of the parietal and frontal lobe known to be endowed with the mirror mechanism [43] . On the other hand, other authors reported repetition suppression of BOLD responses in the human dorsal stream, either by presenting object-directed hand actions [28] , [39] , [40] , by showing static pictures describing an object as well as an action [38] or by involving subjects in simulated social interactions in the scanner against a videotaped opponent (the ‘rock-paper-scissor’ game) [31] . Many of the fMRI studies on action observation observed repetition suppression not only in the premotor cortical region thought to accommodate a human mirror neuron mechanism, but in addition in a variety of other visual and visuomotor areas, usually not implicated in mirror neuron mechanisms. As stressed by Bartels et al. [44] , the locus of adaptation is difficult to assess in the case of multiple inputs to a given area, as in the case of premotor cortex. Thus, it seems plausible that the fMRI adaptation effects observed in premotor cortex might actually reflect information encoded elsewhere in cortex and propagated to the area thought to be part of the mirror neuron system. The discrepancy between BOLD responses showing repetition suppression and the electrophysiological signatures of information processing in area F5 disappears if one considers our finding that the LFPs evoked by action observation exhibited significant repetition suppression. It is now widely accepted that the BOLD signal is better correlated with the synaptic activity reflected by the LFPs rather than with the action potentials fired by neurons [44] , [45] , [46] . Afferents impinging on neurons in a given cortical area make a substantial contribution to the overall synaptic activity. In other words, the BOLD signal is significantly influenced by the input to an area, which is not to say that local processing cannot make a contribution. Hence, it seems conceivable that repetition suppression of the input may be responsible for repetition suppression of the BOLD signal. This could occur, for example, in visual neurons of the superior temporal sulcus region coding observed hand motor acts [47] or in inferotemporal cortical neurons sensitive to object properties. When trying to relate BOLD repetition suppression to changes of spiking activity, usually several possible mechanisms, namely neuronal fatigue, response facilitation and response sharpening as well changes in visual expectations are discussed [20] . Our data clearly show that none of these mechanisms is compatible with the properties of F5 mirror neurons, the simple reason being that the population of F5 mirror neurons do neither exhibit repetition suppression nor change their timing with the repetition (as assumed by the ‘facilitation model’). Why should the discharge of F5 mirror neurons not simply follow the input as thought to be reflected in both the LFPs and the BOLD signal and show repetition suppression as well? The speculative answer we would like to suggest assumes that our sample of mirror neurons is dominated by pyramidal neurons, that is, cortical output neurons, whose share in the mammalian cerebral cortex is usually estimated to be on the order of 70–80%(ref. 48 ). Next, assuming a balanced network in which excitatory and inhibitory activities compensate each other [49] , we speculate that adaptation of direct input to pyramidal neurons might actually be compensated by adaptation of inhibition provided by cortical interneurons, the latter assumed to faithfully transmit the adaptation of their input. Actually, if the adaptation of interneuron-based inhibition overweighed the adaptation of the direct input to pyramidal neurons, an enhancement of the responses of pyramidal neurons would result. Again assuming that our sample is dominated by pyramidal neurons, this would explain our finding of an increase of the responses with repetition. Conversely, shifting the balance in favour of the direct input to pyramidal neurons, adaptation of the action potential output should result as found in a number of studies of visual cortex. However, why should the balance of excitatory/inhibitory inputs differ between mirror neurons and neurons in visual cortex? Our again speculative answer is that this may be a consequence of subtle architectural differences between visual and premotor cortex [50] . These considerations are speculative indeed. Their purpose can only be to demonstrate that a unifying physiological mechanism is in principle able to predict qualitatively different neuronal responses to repeated stimulation. Alternatively, action potential firing may simply be less sensitive to repetition suppression than LFPs. Nevertheless, this speculation has the disadvantage that it should be a peculiar characteristic of single neurons in the premotor cortex as it cannot easily account for the observation of repetition suppression of action potential firing in other visual [1] , [2] , [3] , [4] , inferior [5] , [6] , [7] , [8] , [9] , [10] , [11] , [12] , [13] , [14] , [15] and medial temporal cortical areas [16] , [17] , [18] . The bottom line is that a simple one-to-one relationship between repetition suppression of BOLD responses and action potentials firing cannot be taken for granted. In other words, conclusions on the output of a cortical area based on the fMRI repetition paradigm should be drawn only very cautiously. Subjects and recording methods The experiments were carried out on two male rhesus monkeys ( M. mulatta ). During the experiments, the monkeys sat comfortably in a primate chair. The movements of the left arm were restrained gently by a comfortable gauze bandage, whereas the right arm was free to move. The movements of the monkey’s head were restrained painlessly by means of a head holder attached to the skull and eye position was monitored continuously using chronically implanted search coils. We monitored the monkey behaviour online by means of two infrared cameras; one was directed at the monkey’s body (to detect possible body movements), the other one delivered a close up of the monkey’s face. Surgery and recording methods followed previous descriptions [36] , [37] . All animal preparations and procedures fully complied with the NIH Guide for Care and Use of Laboratory Animals, and were approved by the local ethical committee (Regierungspraesidium Tuebingen). Motor and visual tasks Both the motor and the visual task as well as the apparatus and the control were the same as the one used in previous experiments [36] , [37] . In brief, both monkeys were trained to grasp and lift in darkness one of three small metallic objects placed at defined locations within their workspace. Each individual object afforded only one of three possible grips: power grip, precision grip and finger prehension. The monkeys were trained to grasp, with the appropriate grip, the object that was cued by switching on an LED positioned immediately in front of the object. To test the properties of visual responses to filmed motor acts, neurons were tested by showing previously taped motor acts on an LCD screen placed at a distance of 40 cm in front of the monkey. The visual paradigm ( Fig. 1a ) consisted of a sequence of: (1) a red spot (0.25 deg × 0.25 deg) displayed for a variable time (1,000–2,500 ms); (2) a movie that was presented for a duration of 5,000 or 10,000 ms with a size of about 15 deg × 18 deg visual angle (see its description below); (3) a spot (0.25 deg × 0.25 deg) that was presented for a variable time (500–1,500 ms) with two different colours (red—followed by a small reward, green—followed by a large reward). As long as the spot was visible (first and third phase of the sequence), the monkey was required to keep its eyes within a fixation window of 3° × 3° centred on the spot. During presentation of the movie (phase 2), the fixation window was enlarged such as to cover the whole area of the movie. The monkey was rewarded with a drop of water/juice at the end of a trial, that is, after the offset of the second fixation spot (third phase), if it had met the fixation requirements. Movies, as well as the other visual stimuli, were presented by custom-made real-time software ( http://nrec.neurologie.uni-tuebingen.de ) with a refresh rate of 60 f.p.s. Visual stimuli Actions performed by a human hand were recorded by means of a Canon XL1-S video camera at 25 frames per seconds with a resolution of 640 × 480 pixels in a non-compressed format. The camera was placed above the left shoulder of the actor while he used the right hand to reach and manipulate the object. The recorded video sequences were edited (Matlab) to generate video clips with a duration of 5 s (125 frames) or 10 s (250 frames) with a resolution of 320 × 250 pixels in a non-compressed format. Hand and object were segmented based on colour information from the black background. Pixel values corresponding to the remaining background were substituted by homogeneous Gaussian noise estimated from the original background to ensure a homogenous background. Each frame was finally smoothed with a normalized Gaussian kernel function (with s.d. 1 pixel). In Experiment 1, the movie started with the presentation of an isolated object (a red pepper) for about 840 ms. After this presentation, a hand entered the scene, reaching the object, holding it for about 200 ms, then withdrew from it and finally left the scene. These motor acts lasted for about 1,360 ms. After about 640 ms in which the isolated object was shown, the identical motor act was repeated ( Fig. 2a ). To reduce the role of prediction of the upcoming stimulus, in some sessions the action was presented without repetition or the time interval between the two movies was varied by randomly choosing intervals of 360, 640 or 1,080 ms. In this case, only trials with repeated actions with the standard interval of 640 ms were considered for later analysis. The trials, in which the two actions movies, whose effects on the neuronal discharge were studied, were presented interleaved with other trials (between 6 and 12) showing different types of object-related motor acts, with and without repetition within a given trial. In Experiment 2, after the presentation of the isolated object for 840 ms, the same action was repeated four times. Between consecutive actions, the isolated object was shown for about 640 ms. Data analysis Data were analysed using custom software written in Matlab (Mathworks Inc.). Neurons were only considered for data analysis if they had been recorded long enough to achieve a minimum of eight valid trials for each condition in both the motor and the visual tasks. Eye movements were stored continuously during experimental sessions at a sampling rate of 12.5 kHz, offline down-sampled to a frequency of 125 Hz and filtered with a Savitzky–Golay method with a span of 12 data points for further analysis. Analysis of the motor responses followed the same procedure already described [36] , [37] . To quantify the visual responses to filmed actions we computed average discharge rates separately for the different grip phases in the movie (four phases: baseline, approaching, grasping, withdrawing). The baseline activity was computed as the average discharge rate in the interval between 200 and 840 ms after the beginning of the movie, that is, while the image of a stationary pepper without hand was presented. Only neurons showing significant activity, with respect to baseline, in at least one of the other phases were classified as responsive to that condition (Kruskal–Wallis, P <0.05, Bonferroni corrected for multiple comparisons). The adaptation index of the average activity of an individual neuron was computed by taking the difference between the average activity during the whole period of presentation of the first action and the average activity during the whole period of presentation of the second action and then normalizing this difference by dividing it by the average activity associated with the first presentation. The adaptation index of the maximum was determined by measuring the size of the peak discharge rate after smoothing the spike activity with a Gaussian kernel of 100 ms s.d. for each presentation period. The values obtained were rectified (to account for occasional discharge rate decreases) and baseline corrected. The adaptation index was then calculated by taking the difference of the resulting values for the two presentations, divided by the value for the first presentation. A response related to the expectation of reward was detected by comparing (sign-rank test) the average discharge rate for the 500 ms preceding the presentation of the first action stimulus with the average discharge rate in the period from 200 to 700 ms after the termination of the second action stimulus. If a neuron showed a significant change ( P <0.05), it was interpreted as being influenced by the expectation of reward. This was the case in 35% of the recorded neurons. LFPs data were obtained by subsampling the raw signal at 500 Hz and by filtering it with a band pass filter between 1 and 100 Hz (two-pole Butterworth). After filtering, data were transformed into z -scores to account for differences in the gain of the signal recorded from different electrodes. Records exceeding +/−2 s.d. of the mean activity, exceeding a threshold of two s.d. of the joint probability (EEGlab toolbox [51] ) or exceeding a threshold of two s.d. of the kurtosis of the activity (EEGlab toolbox [51] ) were taken as artifacts and discarded. Data were aligned with the same triggers used to align action potentials. Each recording session available in principle contributed to the population analysis. However, in an attempt to avoid a bias for the sites explored more frequently, a particular site contributed with an averaged based on all session that had involved that site (reduced set of recording sites). In addition to the adaptation index, we calculated an adaptation contrast using the following formula: where X 1 is the lfp signal recorded during the presentation of the first action and X 2 is the lfp signal recorded during the presentation of the second action. How to cite this article: Caggiano, V. et al. Mirror neurons in monkey area F5 do not adapt to the observation of repeated actions. Nat. Commun. 4:1433 doi: 10.1038/ncomms2419 (2013).